Blending of animal colour patterns by hybridization Biologists have long been fascinated by the amazing diversity of animal colour patterns. Despite much interest, the underlying evolutionary and developmental mechanisms contributing to their rich variety remain largely unknown, especially the vivid and complex colour patterns seen in vertebrates. Here, we show that complex and camouflaged animal markings can be formed by the 'blending' of simple colour patterns. A mathematical model predicts that crossing between animals having inverted spot patterns (for example, 'light spots on a dark background' and 'dark spots on a light background') will necessarily result in hybrid offspring that have camouflaged labyrinthine patterns as 'blended' intermediate phenotypes. We confirmed the broad applicability of the model prediction by empirical examination of natural and artificial hybrids of salmonid fish. Our results suggest an unexplored evolutionary process by means of 'pattern blending', as one of the possible mechanisms underlying colour pattern diversity and hybrid speciation. Animals have various colour patterns on their body surfaces, providing vivid examples of the enormous biodiversity [1] , [2] . Recent studies have revealed the evolutionary and developmental mechanisms underlying the diversity in some colour patterns, such as black spots on insect wings [3] , [4] . These spot patterns seem to be formed from genetically encoded blueprints: spatially restricted expression of certain genes that are controlled by multiple cis -regulatory elements [4] , [5] . Thus, these patterns can be thought of as 'fixed' traits within each species, and, therefore, a hybrid offspring between species that have different spot patterns will have a superimposed image of the parent patterns [6] as a natural consequence of the 'sum' of two different cis -regulatory element sets from both parents. On the other hand, some other colour patterns observed in nature (especially of vertebrates) seem to be more complicated and 'flexible'. For example, the markings of leopards or whale sharks are not fixed within species but rather specific to each individual: the exact position of each spot or stripe is variable and there are subtle differences within a species, or even between the left and right sides of an individual. Moreover, colour patterns of some animals are dynamically and autonomously rearranged to resolve pattern inconsistency caused by body growth or artificial disturbance [7] , [8] , indicating the flexible property of underlying mechanisms. Multiple different factors have been identified that affect such 'flexible' colour patterns [9] , [10] , indicating the potentially quantitative nature of these traits. As for quantitative traits, hybrid offspring generally have intermediate phenotypes, which can be readily predicted if the traits are defined and measured as one-dimensional morphological variables (for example, length and/or number of body parts [11] , [12] , overall colour tone of the body [13] ). However, it is unclear whether the flexible two-dimensional colour patterns also produce intermediate forms, and, if so, what pattern is the precise 'intermediate' between similar but different colourations, such as 'white spots on a black background' and 'black spots on a white background'. So far, many attempts have been made to reproduce flexible colour patterns in animals by using mathematical modelling. Among them, a specific class of reaction-diffusion (RD) systems [14] have been frequently used, which can account for many complex biological patterns [15] , [16] on the basis of a simple rule: local self-activation and long-ranging inhibition [17] . The RD model also provided an unexpected prediction for the dynamic processes of colour pattern rearrangement on actual animals [7] , [8] , implying that it captures the very essence of the flexible colour pattern formation mechanisms. Here, we use the RD model for an ' in silico hybridization' experiment to explore the possible intermediate forms of the flexible two-dimensional traits, and demonstrate that, supported by the examination of actual hybrid animals, a complex and camouflaged pattern can be formed by 'blending' a set of simple spot patterns. In silico hybridization predicts camouflaged colour patterns By the gradual modulation of a certain parameter in the RD model equations, various two-dimensional patterns can be reproduced, including spot patterns and inverse spot patterns ( Fig. 1 ). Assuming that one continuous parameter is determined by multiple 'genetic loci' (that is, polygenic inheritance) and that any 'individuals' having different parameter values can be 'crossed' with each other, the resultant 'hybrid' will have a parameter value that is intermediate between those of the 'parents'. On the basis of the simulation results, we focused on the following point: regardless of the model equations and parameters chosen for the simulation, if there are two parameter regions that yield spot and inverse spot patterns, an intermediate region must exist in which camouflaged 'labyrinthine' patterns will arise ( Fig. 1 ). This type of pattern transition has been well recognized among theorists [15] , and when this is applied to the biological context, the following non-trivial prediction can be derived: if an animal having 'light spots on a dark background' is crossed with another animal having 'dark spots on a light background', the resultant hybrid offspring will necessarily have 'labyrinthine' patterns. 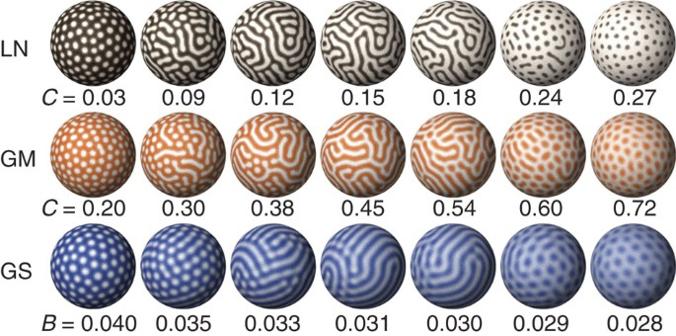Figure 1: Two-dimensional patterns generated by numerical simulations. In each model, gradual modulation of one parameter value (indicated below each sphere) can cause pattern changes from spots (left most) to inverse spots (right most). Intermediate regions always appear as labyrinthine stripe patterns. Each colour represents the concentration of the core factor in each model (brown: activator in the linear model, LN; orange: activator in the Gierer–Meinhardt model, GM; blue: autocatalytic enzyme in the Gray–Scott model, GS. Lighter colour indicates higher concentration). The equations and details for simulations are provided in the Methods section. Figure 1: Two-dimensional patterns generated by numerical simulations. In each model, gradual modulation of one parameter value (indicated below each sphere) can cause pattern changes from spots (left most) to inverse spots (right most). Intermediate regions always appear as labyrinthine stripe patterns. Each colour represents the concentration of the core factor in each model (brown: activator in the linear model, LN; orange: activator in the Gierer–Meinhardt model, GM; blue: autocatalytic enzyme in the Gray–Scott model, GS. Lighter colour indicates higher concentration). The equations and details for simulations are provided in the Methods section. Full size image To test this prediction, we investigated the colour patterns of actual hybrid animals. The white-spotted charr ( Salvelinus leucomaenis ) and masu salmon ( Oncorhynchus masou masou ) are both salmonid fish with fluvial forms (as well as sea-run forms) seen in Japanese rivers. The former has light spots and the latter has dark spots on the sides of their bodies ( Fig. 2a,b ). They usually live in different habitats (the former lives more upstream), yet natural hybridization occasionally occurs between these species [18] . We observed natural and artificial hybrid individuals, all of which showed peculiar vermiculated stripe patterns, or labyrinthine patterns, in very good accordance with the simulation results ( Fig. 2c,d ). 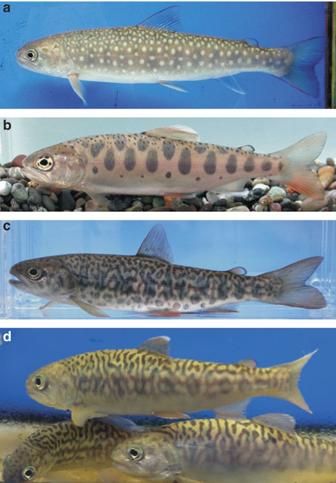Figure 2: Body patterns of salmonid fish. (a) White-spotted charr (S. leucomaenis), (b) masu salmon (O. masou masou) and (c) their natural and (d) artificial intergeneric hybrids. Peculiar labyrinthine patterns are seen in all the hybrids. Figure 2: Body patterns of salmonid fish. ( a ) White-spotted charr ( S. leucomaenis ), ( b ) masu salmon ( O. masou masou ) and ( c ) their natural and ( d ) artificial intergeneric hybrids. Peculiar labyrinthine patterns are seen in all the hybrids. Full size image Colour pattern dynamics in multidimensional trait space In the model organism zebrafish, multiple factors have been identified that affect their stripe colour pattern in different ways [9] , [10] , [19] , [20] , [21] , [22] . The in silico hybridization can also be extended naturally to a multidimensional parameter space, in which multiple parameters of a model can be manipulated simultaneously, but independently ( Fig. 3 ). In this situation, pattern modification caused by a change in one parameter could be largely compensated for by other parameters. 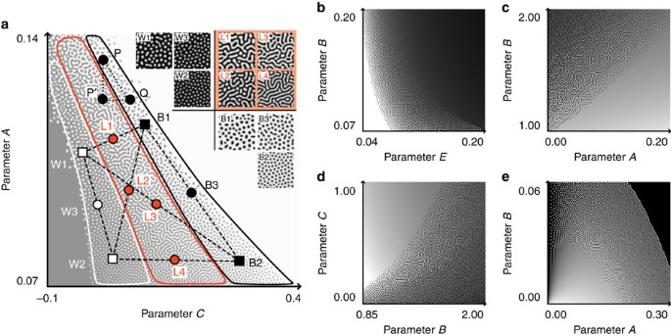Figure 3: 'In silicohybridization' in the two-dimensional parameter space. (a) Pattern dynamics in the linear model RD system. Each point (x, y) represents a parameter set (C=x,A=y) for the model equations. The labyrinthine pattern zone (outlined by the red border) lies between the white spot zone (white bordered) and the black spot zone (black bordered). Broken line segments joining the coloured squares (W1–2 and B1–2) denote 'in silicohybridization' between distinct parameter sets ('genotypes'). The midpoints of these segments (coloured circles; W3, B3 and L1–4) correspond to the 'hybrids'. The colour patterns calculated using the parameter sets of the indicated points are shown in the insets. (b–e) Pattern dynamics with various parameter sets and models. (b) Linear model, (c,d) the Gierer–Meinhardt model and (e) the Gray–Scott model. For instance, in the two-dimensional parameter space depicted in Figure 3a , a change in the pattern because of the shift of parameter A (point P to P′) can be cancelled out by the counteractive shift of parameter C (point P′ to Q), which results in similar black spot patterns (P and Q). Under such conditions, the similarity or identity of colour pattern phenotypes does not necessarily imply the complete concordance of underlying parameter sets. On the contrary, in the case of actual animals, it is reasonable to expect certain differences in the 'parameter sets' (or genotypes) between different species, even though they have similar patterns (for example, W1 versus W2 and B1 versus B2 in Fig. 3a ). However, from the in silico hybridization, we also predicted that any combination between 'white spots' and 'black spots' species, regardless of the underlying parameter sets, would always give birth to hybrid offspring with labyrinthine patterns ( Fig. 3a , L1–4). In contrast, crossing within 'white spots' species or within 'black spots' species would never cause major changes in the colour patterns of their progeny ( Fig. 3a , W3 and B3). Similar results can also be obtained with other parameter sets or models ( Fig. 3b–e ). Figure 3: ' In silico hybridization' in the two-dimensional parameter space. ( a ) Pattern dynamics in the linear model RD system. Each point (x, y) represents a parameter set ( C =x, A =y) for the model equations. The labyrinthine pattern zone (outlined by the red border) lies between the white spot zone (white bordered) and the black spot zone (black bordered). Broken line segments joining the coloured squares (W1–2 and B1–2) denote ' in silico hybridization' between distinct parameter sets ('genotypes'). The midpoints of these segments (coloured circles; W3, B3 and L1–4) correspond to the 'hybrids'. The colour patterns calculated using the parameter sets of the indicated points are shown in the insets. ( b – e ) Pattern dynamics with various parameter sets and models. ( b ) Linear model, ( c , d ) the Gierer–Meinhardt model and ( e ) the Gray–Scott model. Full size image Evidence supporting these predictions was found in earlier studies. In the 1970s, Suzuki and Fukuda [23] conducted a comprehensive and exhaustive analysis of artificial hybridizations among salmonid fish (62 heterologous combinations in total), aiming to develop suitable hybrid species for inland fish farming. We reexamined their data, focusing on the colour patterns of the hybrids ( Fig. 4 ). According to their experiments, viable interspecific hybrids within the genus Salvelinus (2 combinations, 30 individuals each) showed 'light spots on dark background', as seen in their parents ( Fig. 4a ), and interspecific and intergeneric hybrids of the genera Oncorhynchus and Salmo (4 combinations, 11–30 individuals each) showed 'dark spots on light background', similar to their parents ( Fig. 4d ). On the other hand, all viable intergeneric hybrids between Salvelinus (light spots) and Oncorhynchus or Salmo (dark spots) (8 combinations, 12–30 individuals each) exhibited labyrinthine colour patterns ( Fig. 4b,c ). Compared with the simple spot patterns of the parent species, the labyrinthine patterns of the hybrids showed higher complexity in their shape, although they are intermediate in their overall colour tone ( Fig. 4e ). The same or similar examples have also been repeatedly reported among Japanese and North American species of the family Salmonidae [18] , [24] , [25] . All these observations are entirely consistent with our predictions derived from the ' in silico hybridization' using RD models ( Fig. 4e ). 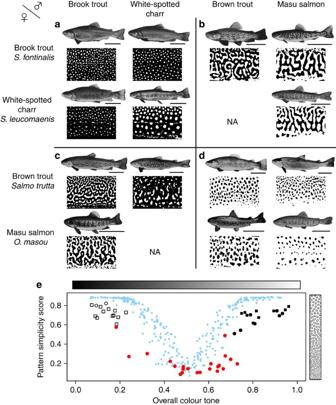Figure 4: Pattern variations in actual hybrid animals. Artificial hybrids between female (rows) and male (columns) salmonid species and the binarized images of their body patterns (taken fromFig. 2and study by Suzuki and Fukuda23). Interspecific hybrids within the 'white spots' group (a) have white spots. Intergeneric hybrids between the 'white spots' group and the 'black spots' group mostly display labyrinthine patterns (b,c). Interspecific and intergeneric hybrids within the 'black spots' group (d) have black spots. Scale bar, 10 cm. (e) Quantification of colour patterns. The complexity of each colour pattern (lower score means higher complexity; seeMethodssection) is plotted against the overall colour tone of the pattern (defined as the ratio of white area). Hybrids between 'white spots' species and 'black spots' species (red circles) have more complex patterns than those of the parent species (white or black squares), whereas they have intermediate values for the overall colour tone. Hybrids within the 'white spots' group (white circles) and within the 'black spots' group (black circles) have similar values for both indices to the parents. Blue dots denote calculated patterns using the RD model. Figure 4: Pattern variations in actual hybrid animals. Artificial hybrids between female (rows) and male (columns) salmonid species and the binarized images of their body patterns (taken from Fig. 2 and study by Suzuki and Fukuda [23] ). Interspecific hybrids within the 'white spots' group ( a ) have white spots. Intergeneric hybrids between the 'white spots' group and the 'black spots' group mostly display labyrinthine patterns ( b , c ). Interspecific and intergeneric hybrids within the 'black spots' group ( d ) have black spots. Scale bar, 10 cm. ( e ) Quantification of colour patterns. The complexity of each colour pattern (lower score means higher complexity; see Methods section) is plotted against the overall colour tone of the pattern (defined as the ratio of white area). Hybrids between 'white spots' species and 'black spots' species (red circles) have more complex patterns than those of the parent species (white or black squares), whereas they have intermediate values for the overall colour tone. Hybrids within the 'white spots' group (white circles) and within the 'black spots' group (black circles) have similar values for both indices to the parents. Blue dots denote calculated patterns using the RD model. Full size image We showed theoretically and empirically that camouflaged labyrinthine patterns can be formed by the 'blending' of simple spot patterns. Besides the salmonid hybrids, many organisms have labyrinthine patterns in nature (particularly among teleosts), and some of them are closely related to other species with spot/inverse spot patterns (for example, vermiculated spinefoot, Siganus vermiculatus and marine pufferfish, Takifugu exascurus ). We speculate that at least some of the organisms with labyrinthine patterns may have resulted from the 'pattern blending' mechanism proposed here. Several cases have been reported in which previously recognized distinct species of marine fish were later identified as the F1 hybrid of other species [26] . Ongoing advances in comparative genomics of marine species may accelerate the detection of more such hybrids. Furthermore, we considered another possibility that labyrinthine organisms may have evolved as species of hybrid origins, rather than be mere F1 hybrids. Accumulating evidence indicates that natural hybridization can contribute to the evolutionary process of animal speciation [6] , [27] , [28] , [29] , [30] , [31] . The labyrinthine phenotype we described here may be another conspicuous example of such cases, which fulfils the requirements for hybrid speciation. The complex and camouflaged pattern differs markedly from either pattern of the parent species and therefore is possibly more advantageous in some environments. This means that a natural 'intermediate' state of a two-dimensional quantitative trait can coincidentally represent a 'transgressive' phenotype, even without any special genetic mechanisms (a novel mode of 'transgressive segregation' [32] ). At the same time, animal markings are known to be frequently used as visual cues for species recognition and mate choice [33] , [34] , including the form of assortative preferences [6] . In cases in which colour patterns (but not mere colour) are critically involved in assortative mating, a group of individuals with the same or similar 'blended' patterns will be prezygotically isolated from the parent species; thus, they may evolve as a distinct lineage of hybrid origin. For a comprehensive appreciation of biodiversity, animal colour patterns are undoubtedly one of the most attractive targets. Further understanding of their diversity requires detailed analyses of the molecular and cellular mechanisms of the pattern formation processes. Comparative genomic studies among related species with divergent colourations [35] , [36] will also have an important role. In addition, the 'pattern blending' model we proposed here may provide a platform for the integrated understanding of the flexible (and often reticulated) patterns on animal body surfaces and their (possibly reticulate) evolutionary processes. Computer simulations Equations used for RD systems [14] can be generally described as where u and v are the concentrations of hypothetical factors, f and g are the reaction kinetics and D u and D v are the hypothetical diffusion coefficients (or their mathematical equivalents) for u and v , respectively [15] , [37] . The reaction rate R was introduced for convenience of parameter adjustment. The reaction kinetics and parameters used for each simulation are as follows: The linear model: [14] where A =0.08 ( Fig. 1 ), B =0.08, D =0.03, E =0.10, F =0.12, G =0.06, D u =0.5 ( Fig. 1 ) and 1.0 ( Fig. 3 ), D v =10.0 ( Fig. 1 ) and 20.0 ( Fig. 3 ), R =20.0, and the lower and upper limits for the synthesis rates of u ( Au + Bv + C ) and v ( Eu−F ) are set as where synU max =0.23 and synV max =0.50. The Gierer–Meinhardt model: [17] where A =0.08, B =1.5, D u =0.5 ( Fig. 1 ) and 1.0 ( Fig. 3 ), D v =10.0 ( Fig. 1 ) and 20.0 ( Fig. 3 ), and R =1.0 ( Fig. 1 ) and 0.2 ( Fig. 3 ). The Gray–Scott model: [38] where A =0.03, D u =0.5 ( Fig. 1 ) and 1.0 ( Fig. 3 ), D v =10.0 ( Fig. 1 ) and 20.0 ( Fig. 3 ), and R =8.0 ( Fig. 1 ) and 2.0 ( Fig. 3 ). Simulations were carried out on two-dimensional square grids ( Fig. 3 ) or on evenly distributed cells on a sphere ( Fig. 1 ). The field sizes were 1,024×1,024 ( Fig. 3 ), 128×128 ( Fig. 3a insets) and 20,000 cells ( Fig. 1 ). The initial conditions included random patterns of u and v . The Neumann boundary condition was used in Figure 3 , and periodic boundary condition in Figure 3a insets. The time step for all simulations was set as d t =0.01. Calculations were performed with 20,000 ( Fig. 1 , the linear model and the Gierer–Meinhardt model), 50,000 ( Fig. 3a,b,e ), 80,000 ( Fig. 3c,d ) and 100,000 ( Fig. 1 , the Gray–Scott model) iterations. The POV-Ray is a computer program. was used for rendering ( Fig. 1 ). Fortran and MATLAB codes are available from the authors on request. Natural and artificial hybrids of salmonid fish All animal experiments were conducted in accordance with the institutional guidelines of Osaka University and Sapporo Salmon Museum. A specimen of a natural hybrid of salmonid fish was collected in 2005 from Teine, Sapporo. The external characters of the hybrid specimen were intermediate between those of the two native salmonids, S. leucomaenis and O. masou masou . Artificial hybridization between S. leucomaenis and O. masou masou was conducted in 2006 at the Sapporo Salmon Museum, Sapporo. Eggs were stripped from two S. leucomaenis females and mixed with sperm obtained from two O. masou masou males. Water temperature was maintained at about 10 °C. Hybrids were observed 33 months after hatching. Crossing between female O. masou masou and male S. leucomaenis was unsuccessful, as reported previously [39] . Quantification of colour patterns Colour pattern complexity and overall tone were quantified from binarized images using the OpenCV library. The pattern simplicity score (PSS) is defined as the area-weighted mean isoperimetric quotient of the contours extracted from each image: where is the isoperimetric quotient (or circularity) of each contour, is the area weight, S i and L i are the area and the perimeter of each contour, respectively. The overall colour tone of a pattern is defined and calculated as the ratio of unpigmented area (white pixels in the binarized image). How to cite this article: Miyazawa, S. et al . Blending of animal colour patterns by hybridization. Nat. Commun. 1:66 doi: 10.1038/1071 (2010).